In situobservation of filamentary conducting channels in an asymmetric Ta2O5−x/TaO2−xbilayer structure Electrically induced resistive switching in metal insulator-metal structures is a subject of increasing scientific interest because it is one of the alternatives that satisfies current requirements for universal non-volatile memories. However, the origin of the switching mechanism is still controversial. Here we report the fabrication of a resistive switching device inside a transmission electron microscope, made from a Pt/SiO 2 / a -Ta 2 O 5− x / a -TaO 2− x /Pt structure, which clearly shows reversible bipolar resistive switching behaviour. The current–voltage measurements simultaneously confirm each of the resistance states (set, reset and breakdown). In situ scanning transmission electron microscope experiments verify, at the atomic scale, that the switching effects occur by the formation and annihilation of conducting channels between a top Pt electrode and a TaO 2− x base layer, which consist of nanoscale TaO 1− x filaments. Information on the structure and dimensions of conductive channels observed in situ offers great potential for designing resistive switching devices with the high endurance and large scalability. Resistive random access memory (ReRAM) has attracted considerable attention for next-generation non-volatile memory because of its advantages, including simple structure, scalability and fast switching speed [1] , [2] . In recent years, research on oxide-based resistive switching devices has been motivated by a growing demand for three-dimensional stacking of crossbar arrays [3] because metal oxides are suitable materials for fabricating three-dimensional architectural features without the need for high-temperature processes. Recently, we reported a TaO x -based asymmetric passive switching device with which we successfully localized resistance switching and achieved reliable high-endurance bipolar switching [4] . This device, fabricated in a crossbar array, exhibited stable pulse-switching operation with 10 12 cycle endurance and a sufficient retention time exceeding 10 years at 85 °C. To effectively control the switching characteristics with excellent memory performance, a thorough understanding of the switching behaviour is essential [5] , [6] , [7] , [8] . There have been numerous attempts to identify the origin of resistance changes in various transition metal oxides, thereby understanding the switching mechanism associated with the behaviour of oxygen vacancies [9] , [10] , [11] and with the composition modulation [12] , [13] . However, these microscopic experiments did not provide information on the dynamic process of oxygen-vacancy migration and the resulting physical and chemical changes in conduction channels [14] . Recent advances in electron optics and in situ systems for transmission electron microscope (TEM) have enabled rapid imaging with real-time measurements of electrical properties [15] . Currently, there is growing interest in the direct observation and identification of resistive switching in electrochemical metallization cells through in situ TEM studies [16] , [17] , [18] . However, in the case of valence change memories [5] , the observation and identification of conductive channels under different switching conditions were not reported previously because of difficulties in producing reversible resistive switching inside a TEM [14] . We report herein the first observation and identification of conductive channels in the oxide-based resistive switching device with atomic resolution under different switching conditions using a unique in situ probing technique in conjunction with the high spatial resolution of electron energy loss spectroscopy (EELS). For this work, we successfully produced reversible bipolar resistive switching on an asymmetric Ta 2 O 5− x /TaO 2− x bilayer inside a TEM. Each resistance state (set, reset and breakdown) was confirmed using in situ current–voltage ( I–V ) measurements. Structural characterization of Ta 2 O 5− x /TaO 2− x bilayer A resistive switching device with the structure Pt/SiO 2 (1.5 nm)/Ta 2 O 5− x (10 nm)/TaO 2− x (30 nm)/Pt ( Fig. 1a,b ) was used after the initial electroforming step [19] (see Mehods) for in situ probing experiments. We inserted a thin SiO 2 layer at the Pt/Ta 2 O 5− x interface to reduce switching currents (see Supplementary Fig. S1 ). As reported previously, after the deposition of the TaO 2− x (10 3 ~10 4 Ω) base layer (BL) by a reactive sputtering method [4] , the resistance and thickness of the insulating Ta 2 O 5− x (10 8 ~10 9 Ω) layer were controlled using the plasma oxidation technique. A high-resolution TEM image ( Fig. 1b ) of the Ta 2 O 5− x layer (oxygen exchange layer; OEL) showed brighter contrast than that of the TaO 2− x layer (BL) because of a relatively lower concentration of Ta metal. These two tantalum oxide layers exhibited an amorphous structure. The low-energy EELS [20] spectra taken at the Ta 2 O 5− x layer and the TaO 2− x layer showed the metal Ta concentration more clearly ( Fig. 1c ). Considering the peak centred at 21.3 eV (marked A), which corresponds to the bulk plasmon excitation of metal Ta, it is clear that the TaO 2− x layer had a higher concentration of Ta metal than the Ta 2 O 5− x layer, consistent with the high-resolution TEM image (also see the X-ray photoelectron spectroscopy (XPS) result shown in Supplementary Fig. S2 ). Four other peaks observed in Fig. 1c (marked B, C, D and E) are related to the bulk plasmon excitation of tantalum oxides and indicate the presence of various stoichiometric compositions [21] , [22] in the two layers. To identify the tantalum oxide phases using the bulk plasmon peaks, we simulated a low-loss EELS spectrum because the EELS reference data for various tantalum oxides are not available in the literature. The simulation results using the first-principles method based on density functional theory [23] , [24] , [25] are shown in Fig. 1d . Comparison of calculated ( Fig. 1d ) and experimental ( Fig. 1c ) low-loss spectra shows that the 15.6-eV loss (B), the 25.7-eV loss (C) and the 29.6-eV loss (E) correspond to the bulk plasmon peaks for a mixed valence state of TaO 2 –Ta 2 O 5 , whereas the 8-eV loss (D) is the bulk plasmon peak for Ta 2 O 5 (see curve-fitting analysis in Methods). Thus, the experimental low-loss spectra indicate that the amorphous Ta 2 O 5− x and TaO 2− x layers consisted of Ta, TaO 2 and Ta 2 O 5 phases in full agreement with our previous study [26] , which was successfully carried out by XPS, although the base TaO 2− x layer had a lower concentration of Ta 2 O 5 phase than the Ta 2 O 5− x layer. Additional information on the compositional variation can be found in the O-K edge EELS spectra ( Fig. 1e ) taken from the two layers (OEL and BL), namely, weaker oxygen intensity at the TaO 2− x layer reflects a higher concentration of Ta metal, which is consistent with the low-loss EELS data ( Fig. 1c ). The electrical properties of these tantalum oxides were further investigated in an attempt to identify conductive channels in the Ta 2 O 5− x layer (OEL). The band structure calculations showed that the Ta, TaO and TaO 2 phases are metallic, whereas the Ta 2 O 5 phase is an insulator ( Fig. 1f ). The valence band XPS spectrum of the a -TaO 2− x layer taken after the initial electroforming step shows a strong peak near the Fermi level, E F , indicating that there exist more metallic phases in the BL than in the a -Ta 2 O 5− x layer (see Supplementary Fig. S3 ). Therefore, it is reasonable to conclude that resistance-switching phenomena mainly occur between the top electrode and the a -TaO 2− x layer. 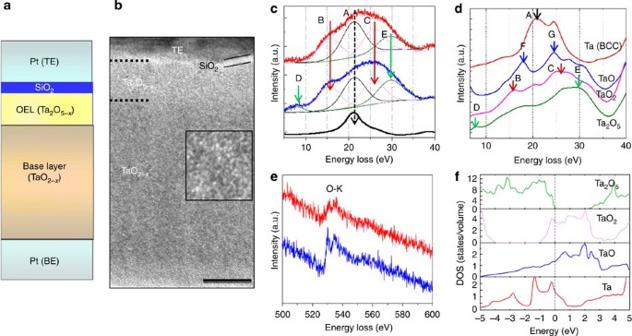Figure 1: A variety of different phases in an asymmetric Ta2O5−x/TaO2−xbilayer structure. (a) Schematic of a resistive switching device with the Pt/SiO2/Ta2O5−x/TaO2−x/Pt structure. (b) Cross-sectional high-resolution TEM image of the Ta2O5−x/TaO2−xbilayer. The inset shows no lattice fringes. Scale bar, 10 nm. (c) Low-energy EELS spectra taken at the Ta2O5−x(blue) and TaO2−x(red) layers as well as at the reference metal Ta (black). Curve-fitting spectra (thin lines) obtained using a minimum number of components based on our reference study and density functional theory calculations are also shown. (d) Simulated plasmon spectra of metal Ta and various tantalum oxides using the first-principles method. (e) Energy loss spectra of O-K edges taken at the Ta2O5−x(blue) and TaO2−x(red) layers. (f) Energy band structure of metal Ta and various tantalum oxides. Figure 1: A variety of different phases in an asymmetric Ta 2 O 5− x /TaO 2− x bilayer structure. ( a ) Schematic of a resistive switching device with the Pt/SiO 2 /Ta 2 O 5− x /TaO 2− x /Pt structure. ( b ) Cross-sectional high-resolution TEM image of the Ta 2 O 5− x /TaO 2− x bilayer. The inset shows no lattice fringes. Scale bar, 10 nm. ( c ) Low-energy EELS spectra taken at the Ta 2 O 5− x (blue) and TaO 2− x (red) layers as well as at the reference metal Ta (black). Curve-fitting spectra (thin lines) obtained using a minimum number of components based on our reference study and density functional theory calculations are also shown. ( d ) Simulated plasmon spectra of metal Ta and various tantalum oxides using the first-principles method. ( e ) Energy loss spectra of O-K edges taken at the Ta 2 O 5− x (blue) and TaO 2− x (red) layers. ( f ) Energy band structure of metal Ta and various tantalum oxides. Full size image Switching behaviour and observation of conducting channels We constructed a ReRAM device that operated inside a TEM using an electron transparent cross-sectional sample of the Pt/SiO 2 /Ta 2 O 5− x /TaO 2− x /Pt structure (cell size of 30 × 30 μm 2 ) to enable real-time observation of the voltage-induced structural changes, in particular, in the conduction channels ( Fig. 2a,b ). The Pt-Ir tip approached the top Pt electrode with the bottom electrode grounded. The switching behaviour of the ReRAM device inside the TEM was confirmed by in situ measurements of the I–V characteristics at various voltages. Indeed, this device sample exhibited reversible bipolar resistance-switching behaviour [4] , [27] between the low-resistance (set) and high-resistance (reset) states by direct current (DC) I–V sweeps ( Fig. 2c ). Most notably, we have first succeeded in demonstrating three consecutive occurrences of the resistive switching in a TEM through the I-V curves of the TaO x -based device (see Supplementary Fig. S4 ). A key conclusion obtained from this multicycle test is that the device resistance following the set process must be controlled with the compliance current (the maximum current through the device) during the set process, because the set resistance has a critical role in the multicycle performance by determining the geometry of the conducting filaments in the TEM device. Initially, the device was in the high-resistance state (HRS). We applied a negative voltage of up to −2.6 V to turn the device into the low-resistance state (LRS) as shown in Fig. 2c . The I–V curve shows that electrical conductivity increases by a factor of ~2,500. A subsequent I–V sweep to a positive voltage of +3.75 V for a very short period of time (10 ms) switched the sample into the HRS, abruptly lowering the conductivity by a factor of ~2,100. The large differences in the current level after set and reset operations were attributed to the fact that many conducting channels contributed to the total current in the ReRAM device [14] . 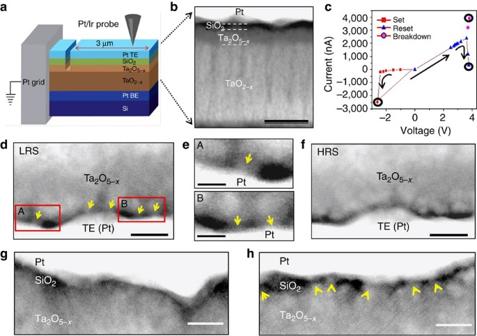Figure 2:In situobservation of the voltage-induced conduction channels. (a) Schematic of thein situexperimental set-up. (b) Cross-sectional HAADF–STEM image when the Pt-Ir tip approached the top Pt electrode. Scale bar, 20 nm. (c) A series ofI–Vmeasurements unambiguously showing reversible bipolar resistive switching. (d–f)In situHAADF–STEM images in LRS (d) and HRS (f), obtained from the blue boxed areas shown inSupplementary Fig. S5. Magnified images of nanoscale channels (e) obtained from the red boxed areas (A and B) ind. Difficulty in observing large areas using the HAADF–STEM imaging mode occurs because of the lower image resolution at the low magnification, which does not allow the exhibition of nanoscale channel formation and annihilation. Scale bars, 5 nm (d,f); 2 nm (e). (g,h) Typical HAADF–STEM images of the Pt/SiO2/Ta2O5−xinterface before (g) and after (h) the electroforming process, showing the incorporation of TaOxinto the SiO2layer after the electroforming process. The contrast fluctuation in the vicinity of the Pt/Ta2O5−xinterface is predominant inh(indicated by yellow arrows), compared to the gradual contrast change ing. Scale bar, 5 nm. Figure 2: In situ observation of the voltage-induced conduction channels. ( a ) Schematic of the in situ experimental set-up. ( b ) Cross-sectional HAADF–STEM image when the Pt-Ir tip approached the top Pt electrode. Scale bar, 20 nm. ( c ) A series of I–V measurements unambiguously showing reversible bipolar resistive switching. ( d – f ) In situ HAADF–STEM images in LRS ( d ) and HRS ( f ), obtained from the blue boxed areas shown in Supplementary Fig. S5 . Magnified images of nanoscale channels ( e ) obtained from the red boxed areas (A and B) in d . Difficulty in observing large areas using the HAADF–STEM imaging mode occurs because of the lower image resolution at the low magnification, which does not allow the exhibition of nanoscale channel formation and annihilation. Scale bars, 5 nm ( d , f ); 2 nm ( e ). ( g , h ) Typical HAADF–STEM images of the Pt/SiO 2 /Ta 2 O 5− x interface before ( g ) and after ( h ) the electroforming process, showing the incorporation of TaO x into the SiO 2 layer after the electroforming process. The contrast fluctuation in the vicinity of the Pt/Ta 2 O 5− x interface is predominant in h (indicated by yellow arrows), compared to the gradual contrast change in g . Scale bar, 5 nm. Full size image We compared the in situ I–V curve ( Fig. 2c ) with the ex situ I–V curve ( Supplementary Fig. S1 ) measured at the cell size of 30 × 30 μm 2 . The ex situ I–V curve of the TaO x -based switching device shows that V set occurs at −1.8 V and V reset at +2.9 V. On the other hand, the in situ I–V curve measured in TEM shows that V set occurs at −2.6 V and V reset at +3.75 V. We believe that the higher switching voltage obtained by the in situ experiment than by the ex situ measurement originates from the contact resistance between the Pt/Ir probe and the top Pt electrode. A large variety of in situ measurements for the switching voltage on other resistive switching memories show the same consequences [16] , [28] . Comparison of the OFF/ON resistance ratio also indicates that the in situ value (~110) is higher than the ex situ value (~90). We expect that this difference can be attributed to the increase of the contact resistance and the oxygen loss in the vacuum of the TEM during the in situ measurements. Nevertheless, the resistance-switching data of the TaO 2− x /Ta 2 O 5− x devices performed in air and vacuum conditions strongly suggest that all oxygen required for resistance switching comes from the tantalum oxide itself [4] . In addition, to minimize the electron-beam heating effect during the in situ TEM experiments, we performed the in situ electrical measurements without electron-beam irradiation. We have obtained high-angle annular dark-field (HAADF) scanning TEM (STEM) images ( Fig. 2d,f ) from the blue boxed areas shown in Supplementary Fig. S5 , which ensures that our in situ HAADF–STEM studies are performed at the same location under different resistance states (LRS and HRS). Comparison of HAADF–STEM images obtained under LRS ( Fig. 2d ) and HRS ( Fig. 2f ) unambiguously exhibited the nanoscale channel formation in the SiO 2 layer (Pt/Ta 2 O 5− x interface); it was ~1.5–2 nm in width and 0.6–1.5 nm in length ( Fig. 2e ). Further, magnified HAADF–STEM images of the boxed area B ( Fig. 2d ) under HRS and LRS demonstrate that tantalum oxide clusters formed after the electroforming process still remained in the SiO 2 layer after the reset operation, and serve to promote formation of the conductive channel for the subsequent set operation ( Supplementary Fig. S6 ). Although we have deposited a 1.5-nm-thick SiO 2 interlayer using a DC magnetron sputtering coupled with plasma oxidation (see Methods), ultrathin regions <1.5 nm (dark region in Fig. 2g ) are non-uniformly distributed because of the rough Ta 2 O 5− x surface. We believe that not only the high electroforming voltage (−3.3 V) but also the rough interface structures result in the incorporation of the tantalum oxide clusters in the SiO 2 layer in the beginning ( Fig. 2h ). Extra HAADF–STEM images give other evidence for the in situ observation of nanoscale channel formation in the different regions (see Supplementary Figs S7 and S8 ). For a nanoscale channel formed in the SiO 2 layer ( Fig. 3a ), we have performed EELS line scans with the corresponding oxygen profiles ( Fig. 3b ). By comparing the oxygen counts in the same channel region after the reset operation, it is clear that the oxygen concentration after the set operation (LRS) is significantly lower than that after the reset operation (HRS), which gives strong evidence for the nanoscale filament formation between a Pt electrode and a Ta 2 O 5− x layer. O-K edge EELS spectra extracted from the line scan in positions E1 and E2 ( Fig. 3b ) clearly reveal the decrease of oxygen intensity after the set operation because of the movement of oxygen-vacancy ( Fig. 3c ). We find, as expected, that a typical low-energy EELS spectrum taken at the nanoscale channel formed in the SiO 2 layer unambiguously exhibits a Ta-O 2,3 edge peak (~39.5 eV) as well as the bulk plasmon peaks of the TaO 1− x phase (18.0 eV (F) and 24.5 eV (G) in Fig. 1d ), whereas the EELS spectrum taken at the SiO 2 barrier layer exhibits a typical bulk plasmon peak for silicon oxide (24.0 eV; Fig. 3d ). As a consequence, the filamentary channels in the SiO 2 layer are composed of the Ta-rich oxide, not silicon oxide. We also quantitatively compared the intensity of HAADF–STEM images shown in Fig. 3a . In a qualitative analysis of the HAADF–STEM images [29] , we found that the intensity ratio of the filamentary tantalum oxide cluster to the SiO 2 area (in LRS) was higher than that of the insulating tantalum oxide cluster to the SiO 2 area (in HRS) because of the formation of Ta-rich filaments relative to the stoichiometric composition (see Supplementary Fig. S9 ). Thus, this contrast difference in the HAADF–STEM images enables us to readily distinguish the presence of tantalum oxides in the SiO 2 layer serving as the conduction channels in LRS. In situ HAADF–STEM images observed during multiple resistive switching cycles (LRS->HRS->LRS) more strongly support our direct observations on the formation and annihilation of conducting channels between a top Pt electrode and a Ta 2 O 5− x BL ( Supplementary Figs S10 and S11 ). 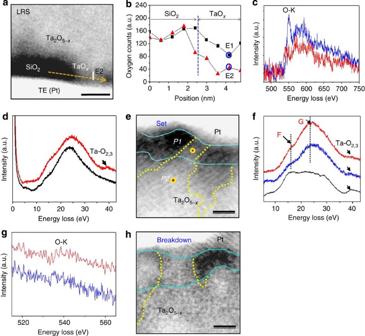Figure 3:Structural and compositional analysis of the nanoscale filament formed in the Pt(TE)/SiO2/Ta2O5−xlayers. (a) Anin situHAADF–STEM image around a channel region obtained under LRS. Scale bar, 2 nm. (b) Horizontal EELS line scans with the corresponding oxygen profiles taken under LRS (red symbol) and HRS (black symbol) moving towards the channel region shown ina. (c) O-K edge EELS spectra extracted from the line scans in positions E1 (blue) and E2 (red). Corresponding position of E2 in the HAADF–STEM image is indicated by a solid white line ina. (d) Comparison of low-loss spectra taken at the nanoscale channel region (red) formed in the SiO2layer and the SiO2region (black) shown ina. (e) An aberration-corrected HAADF–STEM image after the set operation. The region with a higher Ta concentration is brighter. The dotted lines serve as the demarcation line between a Ta-rich area and elsewhere. Scale bar, 1 nm. (f,g) Low-energy EELS spectra (f) and O-K edge EELS spectra (g); with a spatial resolution of 1 nm) taken at the local regions labelledP1(blue) andP2(red) inealong with a low-energy EELS spectrum for the channel region E1 (black) taken under HRS inb. (h) An aberration-corrected HAADF–STEM image after the breakdown operation. Scale bar, 1 nm. Figure 3: S tructural and compositional analysis of the nanoscale filament formed in the Pt(TE)/SiO 2 /Ta 2 O 5− x layers. ( a ) An in situ HAADF–STEM image around a channel region obtained under LRS. Scale bar, 2 nm. ( b ) Horizontal EELS line scans with the corresponding oxygen profiles taken under LRS (red symbol) and HRS (black symbol) moving towards the channel region shown in a . ( c ) O-K edge EELS spectra extracted from the line scans in positions E1 (blue) and E2 (red). Corresponding position of E2 in the HAADF–STEM image is indicated by a solid white line in a . ( d ) Comparison of low-loss spectra taken at the nanoscale channel region (red) formed in the SiO 2 layer and the SiO 2 region (black) shown in a . ( e ) An aberration-corrected HAADF–STEM image after the set operation. The region with a higher Ta concentration is brighter. The dotted lines serve as the demarcation line between a Ta-rich area and elsewhere. Scale bar, 1 nm. ( f , g ) Low-energy EELS spectra ( f ) and O-K edge EELS spectra ( g ); with a spatial resolution of 1 nm) taken at the local regions labelled P1 (blue) and P2 (red) in e along with a low-energy EELS spectrum for the channel region E1 (black) taken under HRS in b . ( h ) An aberration-corrected HAADF–STEM image after the breakdown operation. Scale bar, 1 nm. Full size image To further explore the nature of the conducting channels, we performed detailed structural and compositional analysis of the Pt (TE)/SiO 2 /Ta 2 O 5− x layers. An aberration-corrected HAADF–STEM image obtained after the set operation reveals the nanoscale filament formation in the SiO 2 layer with a Ta-rich cluster (brighter area) in the Ta 2 O 5− x layer being continuously connected to the filament ( Fig. 3e ). To determine the stoichiometry of tantalum oxides in the conducting channel, we have studied low-energy EELS spectra ( Fig. 3f ) and O-K edge EELS spectra ( Fig. 3g ) taken at the local regions labelled P1 (channel formed in the SiO 2 layer) and P2 (Ta-rich cluster in the Ta 2 O 5− x layer), as indicated in Fig. 3e . The bulk plasmon peaks taken at regions P1 and P2 after the set operation are similar to those of the metallic TaO phase (18.0 and 24.5 eV in Fig. 1d ), which was responsible for the dramatic conductivity increase. However, the bulk plasmon peak taken at the position E1 ( Fig. 3b ) reflects the phase transition in the conducting channel from the metallic TaO phase to the insulating Ta 2 O 5 –TaO 2 (coexistence of mixed valence compounds) phase after the Reset operation. The oxygen concentration examined at the two regions ( P1 and P2 ) strongly supports this conclusion ( Fig. 3g ), in full agreement with the EELS line scan data of Fig. 3b . We note here that although the formation and annihilation of conducting channels at the same position as the Ta 2 O 5− x layer have not been fully demonstrated in the aberration-corrected STEM image ( Fig. 3e ) because of the lower sensitivity to the changes in oxygen concentration, the overall agreement with STEM–EELS spectra in the peak positions and relative peak intensities provides clear experimental evidence that the resistive switching mechanism of this tantalum oxide-based device is closely related to the formation of percolating conducting paths from the SiO 2 layer to the TaO 5− x layer through the oxygen-vacancy migration. The current density measured from Fig. 2c reached ~1 × 10 5 A cm −2 . This current density is large enough to induce a thermally assisted electromigration [30] , [31] of oxygen vacancies into the insulating tantalum oxide clusters caused by the accompanying Joule heating effect [32] , [33] at the Pt/SiO 2 interface. This result suggests the possibility that the filamentary channels consisting of the metastable phase TaO 1− x (ref. 34 ) are generated by the local reduction of the tantalum oxide clusters introduced in the SiO 2 layer. We also performed the excess voltage sweep ( V > V set ) over a long period of time (2 s). This process led to the irreversible LRS (breakdown) [35] because of the significant increase in the size and density of conducting channels formed in the SiO 2 layer as well as in the Ta 2 O 5− x layer ( Fig. 3h ). We confirmed the breakdown state by the I–V curve, which indicated that the resistance does not switch back to the reset state ( Fig. 2c ). In our own experience, and according to literature, the breakdown at positive bias is possible if the diffusion of ions assisted by Joule heating has a stronger effect than the drift caused by the applied voltage. All these in situ results strongly support the conclusion that electrical properties are closely correlated to the formation and annihilation of nanoscale channels between a Pt electrode and a TaO 2− x layer. 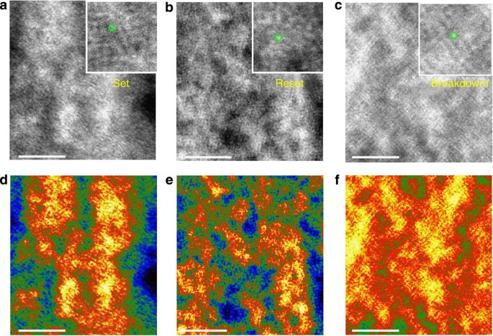Figure 4: Voltage-induced changes in the microstructure ofa-TaO2−xlayer. (a–c) Cross-sectional HAADF–STEM images showing the structural evolution after the set (a), reset (b) and breakdown (c) operations. Bright area: Ta-rich phase (conducting paths), dark area: non-conducting clusters. Insets show the atomic resolution STEM images exhibiting individual Ta atoms (green circles). (d–f) Pseudocolour maps converted from the raw images ofa–c, respectively. Yellow: Ta-rich phase (conducting paths), blue: non-conducting clusters. Bright and yellow regions (ina–f) are regarded as conductive percolation paths. Scale bar, 3 nm (a–f). Figure 4 illustrates typical cross-sectional HAADF–STEM images of the a -TaO 2− x BL taken at the upper part to visualize the voltage-induced variations in the Ta-rich areas during set ( Fig. 4a ), reset ( Fig. 4b ) and breakdown ( Fig. 4c ) operations. To more clearly display the Ta-rich areas indicative of conducting paths in the TaO 2− x BL, the raw STEM image intensities ( Fig. 4a–c ) were converted into colour maps ( Fig. 4d–f ). We confirmed by low-loss EELS analyses that bright and yellow regions ( Fig. 4a–f ) represented conductive clusters consisting of the metallic TaO 1− x phase (see Supplementary Fig. S12 ). At the set state, we observed large conductive clusters that were clearly percolated into the a -TaO 2− x layer ( Fig. 4a,d ). After reset switching, the conductive clusters in the a -TaO 2− x layer became smaller and their percolation paths were partially interrupted ( Fig. 4b,e ). This is similar to the STEM image of the a -TaO 2− x BL in the initial state (see Supplementary Fig. S13 ). After the breakdown operation, the areas of conductive clusters significantly increased as a consequence of almost-filled Ta-rich clusters ( Fig. 4c,f ). Interestingly, the conductive clusters formed after the set operation showed atomic short-range order structure and evolved into a long-range ordering [36] by the excess voltage sweep ( V > V set ) over a long period of time (see Supplementary Fig. S14 ). This observation strongly supports previous results [12] , [37] concerning the crystallization of TiO x and TaO x memristors during the electroforming or switching process. Figure 4: Voltage-induced changes in the microstructure of a -TaO 2− x layer. ( a – c ) Cross-sectional HAADF–STEM images showing the structural evolution after the set ( a ), reset ( b ) and breakdown ( c ) operations. Bright area: Ta-rich phase (conducting paths), dark area: non-conducting clusters. Insets show the atomic resolution STEM images exhibiting individual Ta atoms (green circles). ( d – f ) Pseudocolour maps converted from the raw images of a – c , respectively. Yellow: Ta-rich phase (conducting paths), blue: non-conducting clusters. Bright and yellow regions (in a – f ) are regarded as conductive percolation paths. Scale bar, 3 nm ( a – f ). Full size image The present in situ observations with spatially resolved low-loss EELS analyses and simultaneously measured electrical properties provide insight into the nature of the resistance switching in the asymmetric tantalum oxide-based device. Initially, Ta, TaO 2 and Ta 2 O 5 phases are mixed in the nonconductive a -Ta 2 O 5− x layer. When a negative bias is applied, the tantalum oxide clusters introduced in the SiO 2 barrier layer immediately transform into the TaO 1− x phase, forming filamentary channels by means of oxygen-vacancy migration; at the same time, oxygen vacancies in the a -TaO 2− x layer also diffuse into the a -Ta 2 O 5− x layer, driven by an electric field. A sudden resistance drop occurs when the filamentary channel entirely percolates from Pt top electrode to the a -Ta 2 O 5− x layer ( Fig. 5a ). However, when a positive bias is applied, oxygen ions supplied from the a -Ta 2 O 5− x layer react with the TaO 1− x phase in SiO 2 layer, thereby destroying the conducting channels. At the same time, as oxygen vacancies in the a -Ta 2 O 5− x layer move towards the a -TaO 2− x layer because of the positive bias, the conducting channels (percolation of Ta-rich clusters) formed in the a -Ta 2 O 5− x layer are locally disconnected. Once, the conductive channel breaks in the SiO 2 and a -Ta 2 O 5− x layers by oxygen-ion migration ( Fig. 5b ), the resistance dramatically increases. Percolating clusters, existing at relatively high densities in the a -TaO 2− x layer, also become smaller and are a bit more interrupted than that in the set state. 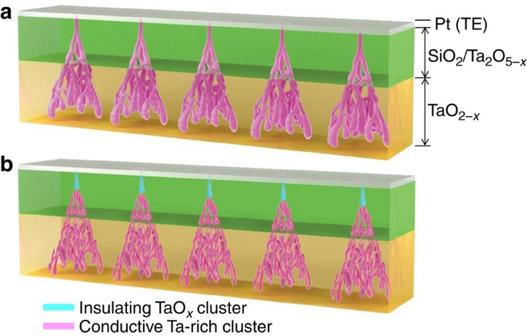Figure 5: Schematic diagrams illustrating resistance-switching mechanism in the Ta2O5−x/TaO2−xdevice. Formation and annihilation of conducting channels during the (a) set and (b) reset states are shown. The pink regions represent conducting clusters consisting of the Ta-rich phases. After reset switching, percolating clusters in thea-TaO2−xlayer become smaller and are a bit more interrupted than in the set state. Figure 5: Schematic diagrams illustrating resistance-switching mechanism in the Ta 2 O 5− x /TaO 2− x device. Formation and annihilation of conducting channels during the ( a ) set and ( b ) reset states are shown. The pink regions represent conducting clusters consisting of the Ta-rich phases. After reset switching, percolating clusters in the a -TaO 2− x layer become smaller and are a bit more interrupted than in the set state. Full size image Oxygen change and number density of nanoscale filaments The Auger electron spectroscopy depth profiles obtained after set and reset operations from the TaO x -based switching device allow us to explain the comprehensive changes of the oxygen concentration in SiO 2 , Ta 2 O 5− x and TaO 2− x layers because of oxygen-vacancy migration ( Fig. 6a ). Comparison of the profiles obtained from the SiO 2 layer to the Ta 2 O 5− x layer unambiguously reveals that the O/Ta ratio measured after the set operation is lower than that after the reset operation. However, the depth profiles measured from the lower part of the TaO 2− x layer yield opposite results. It is clear from these results that oxygen vacancies migrate from the lower part of the TaO 2− x layer, through the Ta 2 O 5− x , to the SiO 2 layer during set operation (under negative bias). From our simulation results using nudged elastic band methods [38] , we have found that the activation energy for charged oxygen-ion migration is much lower at the Ta-rich structure than that at the Ta 2 O 5 structure. Thus, oxygen vacancies in the upper part of the TaO 2− x layer can be accumulated under the set operation by the fast migration of oxygen vacancies from the lower part ( Fig. 6a ). This finding was consistent with the cross-sectional HAADF–STEM images taken in the upper part of the a -TaO 2− x BL under the set ( Fig. 4a ) and reset ( Fig. 4b ) operations; however, the O/Ta ratio measured in the middle part of the TaO 2− x layer remains unchanged irrespective of set and reset operations. Increase of the oxygen concentration in the lower part of the TaO 2− x layer after the set operation was also confirmed by energy-dispersive X-ray spectroscopy line scans ( Supplementary Fig. S15 ). Several studies on films and bulk β-Ta 2 O 5 proved that the mass transport under reducing conditions was predominantly anionic via an oxygen-vacancy mechanism [39] . A recent paper published by Wei et al. [27] also suggested direct XPS evidence for the oxygen migration mechanism in a highly reliable Pt/TaO x /Pt memory cell. 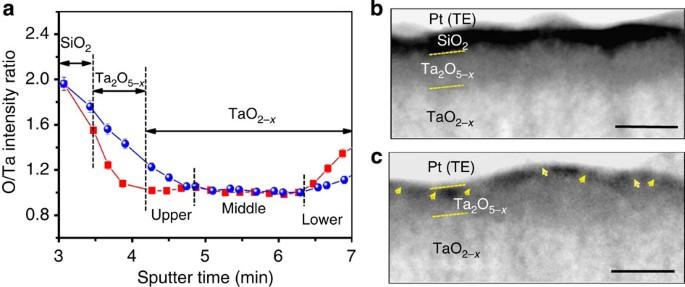Figure 6:Ex situAuger electron spectroscopy (AES) depth profiles and HAADF–STEM images. (a) AES depth profiles of our TaOx-based switching device obtained after set (red) and reset (blue) operations. The error bars of 3% were evaluated by measuring noise signals of O and Ta. (b,c) HAADF–STEM images of the Pt/Ta2O5–xinterface before (b) and after (c) the set operation, showing the formation of many filamentary channels after the set operation. Scale bar, 10 nm. Figure 6: Ex situ Auger electron spectroscopy (AES) depth profiles and HAADF–STEM images. ( a ) AES depth profiles of our TaO x -based switching device obtained after set (red) and reset (blue) operations. The error bars of 3% were evaluated by measuring noise signals of O and Ta. ( b , c ) HAADF–STEM images of the Pt/Ta 2 O 5–x interface before ( b ) and after ( c ) the set operation, showing the formation of many filamentary channels after the set operation. Scale bar, 10 nm. Full size image Comparison of HAADF–STEM images observed before ( Fig. 6b ) and after ( Fig. 6c ) the set operation revealed that many filamentary channels formed at the Pt/Ta 2 O 5− x interface after the set operation whose diameters ranged from 1 to 2 nm, with short distances between the channels. We expect that these filamentary channels in the SiO 2 layer have an important role in opening conducting paths (electric faucet) [40] . The dimensions of the filamentary channels as well as the fractional conducting areas [41] are essential parameters for determining the current level for LRS and HRS and estimating the ultimate packing density of the ReRAM device. The relatively small size and higher density of the filamentary channels formed in the SiO 2 barrier suggest that the memory cell size can be scaled down to 10 nm with a superb uniformity and repeatability. We can consider the total oxide layer as three resistances in a series: R SiOBL , R OEL and R BL for the SiO 2 barrier, oxygen exchange and BLs, respectively, where R SiOBL +R OEL >>R BL in the HRS but R SiOBL +R OEL <R BL in the LRS. In the HRS, the voltage drop occurs across only the SiO 2 barrier and OELs, leading to a localized resistance-switching behaviour. However, in the LRS, the total current flow is controlled by the a -TaO 2− x BL because the resistance value of our device structure (30,000 Ω) is nearly identical to that of the Pt/TaO 2− x /Pt structure (32,500 Ω) in the LRS. It is interesting to note that the results of our in situ experiments reported here suggest an exchange of oxygen vacancies predominantly in the direction of current flow, although a previous EELS analysis on a different tantalum oxide resistive switching system indicated an exchange of oxygen in the direction perpendicular to the current flow due to thermophoresis [12] . Our results are consistent with our previous calculations for the TaO x system [26] and they experimentally confirm the working hypothesis for a large variety of other bipolar switching oxide materials [4] , [5] , [6] , [7] , [8] , [11] . In summary, we have succeeded in reproducing the reversible bipolar resistance-switching behaviour of an asymmetric TaO x -based ReRAM device using an in situ probing method inside a TEM, and we have directly observed the processes of conducting channel formation and annihilation with atomic resolution during the successive resistance switching. With the use of aberration-corrected HAADF–STEM imaging combined with high spatial resolution EELS analysis, we have confirmed that filamentary TaO 1− x channels are created in the SiO 2 barrier layer, and, at the same time, Ta-rich clusters are generated in the a -Ta 2 O 5− x layer owing to the migration of oxygen vacancies, thus achieving perfect conducting nanochannels between a Pt top electrode and a TaO 2− x BL. This resistive switching mechanism provides new insight into the physical and chemical nature of resistance-switching phenomena for oxide systems that have oxygen-poor/-rich bilayer homojunctions. We expect that the in situ experimental technique can further expand its applications in a variety of universal non-volatile memory system. Electroforming Electroforming is the initialization process for resistive switching memory. Electroforming of this ReRAM cell was performed by a DC-negative voltage sweep (−3.3 V), with the compliance current of ~100 μA as demonstrated in Supplementary Fig. S1 . The electroforming process leads to the formation of conducting filaments. The Pt/Ta 2 O 5− x interface after the initial electroforming step becomes conductive by the incorporation of Ta-rich filaments into the SiO 2 layer. Electronic structure calculations Self-consistent calculations of the electronic structures and optical properties based on the full-potential linearized-augmented plane wave method were performed using the WIEN2k package. The exchange and correlation function was treated within the generalized gradient approximation. In this calculation, the space was divided into an interstitial region and into non-overlapping muffin tin (MT) spheres centred at the atomic sites. The valence wave functions inside the spheres were expanded to l max =10 and the wave functions in the interstitial regions were expanded in plane waves with a cutoff of K max =7/ R MT , where R MT denotes the smallest atomic sphere radius and K max is the largest K vector in the plane wave expansion. The R MT were as follows: 1.83(Ta) and 1.62(O) a.u. for Ta 2 O 5 ; 2.25(Ta) and 1.99(O) for TaO; 1.90(Ta) and 1.69(O) for TaO 2 ; and 2.5 for Ta metal. The total density of states and energy loss functions were calculated using summation over 160 k-points within the irreducible Brillouin zone in all cases. All calculations were carried out with relaxation of atomic position until the forces on each atom were below 1 mRy per a.u. The crystalline Ta 2 O 5 exhibited several different polymorphs in crystal structure. For a crystal structure of Ta 2 O 5 , the orthorhombic phase was applied because this structure is reported to be the most stable. For a calculation of Ta bcc metal, intraband transition was considered as well. In the case of a noncubic system, there were three components in ε: ε xx , ε yy and ε zz . The three components of loss functions were calculated and the final loss function was averaged out of the three components. Curve-fitting analysis of low-loss EELS data The curve fitting of Fig. 1c was obtained using a minimum number of components based on our reference study [19] and density functional theory calculations: metallic, monovalent, divalent and pentavalent tantalum oxides. A nonlinear background is assumed and the fitting peaks of the experimental curves are defined by a combination of Gaussian (80%) and Lorentzian (20%) distributions that have fixed FWMH and the energy position of each peak, respectively. An XPS result, obtained by one of authors for the same sample, has shown the presence of Ta 0 , Ta 2+ , Ta 4+ and Ta 5+ at the Ta 2 O 5− x layer [26] . To project this information to our EELS spectra by neglecting the multiplet and charge-transfer effects, a careful peak fitting was performed by using five peaks (marked A, B, C, D and E) assigned to metal-like Ta (A), a mixed valence state of TaO 2 –Ta 2 O 5 (B, C and E), and a Ta 5+ in Ta 2 O 5 (D). The overlapping of peaks and the broadness can be interpreted as a coexistence of mixed valence compounds. Deposition of SiO 2 interlayer A DC magnetron sputtering at room temperature was used for the deposition of a thin Si film (1~2 nm) onto the Ta 2 O 5− x layer. Next, the plasma oxidation of the thin Si film resulted in the insulating SiO 2 interlayer. The thin SiO 2 interlayer at the Pt/Ta 2 O 5− x interface slightly reduced switching currents as shown in Supplementary Fig. S1 . Aberration-corrected STEM/EELS analysis The aberration-corrected STEM/EELS analysis was performed using field-emission TEM (probe-corrected and monochromated FEI Titan) at an accelerating voltage of 300 kV with a high-resolution Gatan imaging filter (GIF Tridiem 865 ER300). The aberration-corrected STEM image was acquired with a convergence angle of 24 mrad. The inner and outer angles of the HAADF detector were 58.5 and 200 mrad, respectively. In addition, the energy dispersion and the collection angle for EELS analysis were 0.02 eV ch −1 and 5 mrad, respectively. The HAADF–STEM image strongly depends on sample thickness and lattice distortion. In the case of the amorphous structure, the effect from static displacement or other strain fields may be neglected; therefore, sample thicknesses and Z -values mostly determine the image contrast. The large HAADF inner angle (58.5 mrad) also eliminates the contribution of static displacement or strain on the image contrast. The sample thickness of the two regions ( P1 and P2 indicated in Fig. 3e ), measured by low-loss EELS using the Fourier-log method, varied within 1%, which was good enough to distinguish between oxygen and Ta (see Supplementary Fig. S16 ). In situ TEM sample preparation We carefully removed the connecting area between the top Pt electrode and the TEM Pt grid by focused ion beam to cut off the current path between the top and bottom electrodes through the Pt grid as shown in Fig. 2a . Thus, the switching active region coincides with the length of the top Pt electrode (~3 μm) being disconnected from the TEM Pt grid. However, we found that there was a decrease in the number density of nanoscale filaments in the region far from the Pt-Ir probe (see Supplementary Fig. S17 ) compared with that in the region near the Pt-Ir probe ( Fig. 6c ). We think that the variation in filament density is because of the difference in stress on the sample region caused by the probe. In situ TEM experiments Specimens for in situ TEM experiments were prepared using the focused ion beam lift-out technique ( FEI, Helios NanoLab 400S). A two-terminal I–V curve was measured using an STM (Nanofactory Instruments AB, ST-1000) installed on a TEM holder serving as a manipulator. The integrity of the contact was constantly monitored during the I–V measurement. We can confirm the sample position during the in situ TEM experiments by observing the position of the Pt-Ir probe placed on the top Pt layer. To minimize the electron-beam heating effect during the in situ TEM experiments, the electron-beam irradiation was blanked during the I–V measurement. How to cite this article: Park, G.-S. et al. In situ observation of filamentary conducting channels in an asymmetric Ta 2 O 5− x /TaO 2− x bilayer structure. Nat. Commun. 4:2382 doi: 10.1038/ncomms3382 (2013).